Expansion of the CRISPR–Cas9 genome targeting space through the use of H1 promoter-expressed guide RNAs The repurposed CRISPR–Cas9 system has recently emerged as a revolutionary genome-editing tool. Here we report a modification in the expression of the guide RNA (gRNA) required for targeting that greatly expands the targetable genome. gRNA expression through the commonly used U6 promoter requires a guanosine nucleotide to initiate transcription, thus constraining genomic-targeting sites to GN 19 NGG. We demonstrate the ability to modify endogenous genes using H1 promoter-expressed gRNAs, which can be used to target both AN 19 NGG and GN 19 NGG genomic sites. AN 19 NGG sites occur ~15% more frequently than GN 19 NGG sites in the human genome and the increase in targeting space is also enriched at human genes and disease loci. Together, our results enhance the versatility of the CRISPR technology by more than doubling the number of targetable sites within the human genome and other eukaryotic species. Genome-editing technologies such as zinc-finger nucleases (ZFNs) [1] , [2] , [3] , [4] and transcription activator-like effector nucleases (TALENs) [4] , [5] , [6] , [7] , [8] , [9] , [10] have empowered the ability to generate targeted genome modifications and offer the potential to correct disease mutations with precision. While effective, these technologies are encumbered by practical limitations as both ZFN and TALEN pairs require synthesizing large and unique recognition proteins for a given DNA target site. Several groups have recently reported high-efficiency genome editing through the use of an engineered type II CRISPR–Cas9 system that circumvents these key limitations [11] , [12] , [13] , [14] , [15] . Unlike ZFNs and TALENs, which are relatively time consuming and arduous to make, the CRISPR constructs, which rely upon the nuclease activity of the Cas9 protein coupled with a synthetic guide RNA (gRNA), are simple and fast to synthesize and can be multiplexed. However, despite the relative ease of their synthesis, CRISPRs have technological restrictions related to their access to targetable genome space, which is a function of both the properties of Cas9 itself and the synthesis of its gRNA. Cleavage by the CRISPR system requires complementary base pairing of the gRNA to a 20-nucleotide DNA sequence and the requisite protospacer-adjacent motif (PAM), a short nucleotide motif found 3′ to the target site [16] . One can, theoretically, target any unique N 20 -PAM sequence in the genome using the CRISPR technology. The DNA-binding specificity of the PAM sequence, which varies depending upon the species of origin of the specific Cas9 employed, provides one constraint. Currently, the least restrictive and most commonly used Cas9 protein is from Streptococcus pyogenes , which recognizes the sequence NGG, and thus, any unique 21-nucleotide sequence in the genome followed by two guanosine nucleotides (N 20 NGG) can be targeted. Consequently, expansion of the available targeting space imposed by the protein component is limited to the discovery and use of novel Cas9 proteins with altered PAM requirements [11] , [17] or pending the generation of novel Cas9 variants via mutagenesis or directed evolution. The second technological constraint of the CRISPR system arises from gRNA expression initiating at a 5′-guanosine nucleotide. Use of the type III class of RNA polymerase III promoters have been particularly amenable for gRNA expression because these short non-coding transcripts have well-defined ends, and all the necessary elements for transcription, with the exclusion of the 1+ nucleotide, are contained in the upstream promoter region. However, since the commonly used U6 promoter requires a guanosine nucleotide to initiate transcription, use of the U6 promoter has further constrained genomic-targeting sites to GN 19 NGG [13] , [18] . Alternative approaches, such as in vitro transcription by T7, T3 or SP6 promoters, would also require initiating guanosine nucleotide(s) [19] , [20] , [21] . To expand the current limitations of CRISPR–Cas9 targeting, we tested whether, instead of U6, we could utilize H1 pol III as an alternative promoter [22] . Specific cleavage by H1-expressed gRNA Because H1 can express transcripts with either purine (nucleotide R) located at the +1 position, we hypothesized that along with the S. pyogenes Cas9, we could expand the CRISPR-targeting space by allowing for cleavage at both AN 19 NGG and GN 19 NGG sites ( Fig. 1a ). To demonstrate site-specific cleavage by H1-expressed gRNAs, we developed a reporter assay to measure CRISPR-mediated cleavage of a green fluorescent protein (GFP) target gene integrated at the AAVS-1 locus in the H7 human embryonic stem cell line (hESC) [23] ( Fig. 1b ). We measured the loss of GFP fluorescence, due to coding sequence disruption, as a proxy for error-prone non-homologous end-joining (NHEJ) frequency; notably, our assay would underestimate NHEJ, as in-frame mutations or indels that do not disrupt GFP fluorescence would not be detected ( Fig. 1b,c ). H7 cells were electroporated with equimolar ratios of Cas9 and gRNA expression plasmids, and cells were visualized for GFP fluorescence after colony formation. In contrast to the negative control electroporation, all gRNA constructs from the U6 and H1 promoters we tested showed a mosaic loss of GFP signals in cells undergoing targeted mutation ( Fig. 1c and data not shown). Quantitation of total cell number with a nuclear stain enabled cell-based analysis of GFP fluorescence by flow cytometry. Although 100% of constructs resulted in NHEJ, as demonstrated by loss of GFP fluorescence, the range of efficiencies varied for both U6 and H1 constructs ( Fig. 1c , right and data not shown). By expressing gRNAs from either the U6 or H1 promoters, this demonstrates that mutagenesis of the GFP gene can occur at GN 19 NGG or AN 19 NGG sites, respectively. 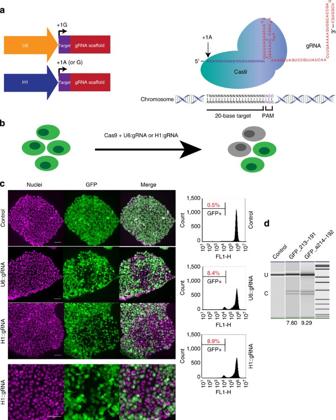Figure 1: Evaluating the ability to direct CRISPR targeting via gRNA synthesis from the H1 promoter. (a) Schematic illustration depicting the gRNA expression constructs. Above, the U6 promoter only expresses gRNAs with a +1 guanosine nucleotide; below, the H1 promoter can drive expression of gRNAs initiating at either purine (adenosine or guanosine) nucleotide. On the right, a cartoon depiction of the Cas9 protein with gRNA targeting genomic sequence AN19NGG. The location of the +1 A is indicated. (b) Schematic overview of the enhanced GFP (eGFP)-targeted disruption assay. eGFP fluorescence is disrupted by CRISPR targeting followed by error-prone NHEJ-mediated repair resulting in frameshift mutations that disrupt the coding sequence, resulting in loss of fluorescence. (c) Microscope images demonstrating successful CRISPR targeting by U6 or H1 promoter-expressed gRNAs. H7 ES cells were stained and colonies were visualized to show nuclei (left, magenta), eGFP fluorescence (middle, green) and merged images (right) indicating areas of GFP fluorescence mosaicism in the colony. To the right is shown the quantification of eGFP fluorescence loss by flow cytometry for the respective constructs. Below is a higher magnification of an H7 colony targeted by an H1-expressed gRNA showing expression mosaicism. Scale bar, 50 μM. (d) Surveyor assay-based quantitation of the frequency of NHEJ. Bioanalyzer gel image depicting control (first lane), U6-expressed gRNA (second lane), H1-expressed gRNA (third lane) and marker (fourth lane). The % indel (as calculated by the fraction of uncut (u) to cut (c) bands) is indicated below. Figure 1: Evaluating the ability to direct CRISPR targeting via gRNA synthesis from the H1 promoter. ( a ) Schematic illustration depicting the gRNA expression constructs. Above, the U6 promoter only expresses gRNAs with a +1 guanosine nucleotide; below, the H1 promoter can drive expression of gRNAs initiating at either purine (adenosine or guanosine) nucleotide. On the right, a cartoon depiction of the Cas9 protein with gRNA targeting genomic sequence AN 19 NGG. The location of the +1 A is indicated. ( b ) Schematic overview of the enhanced GFP (eGFP)-targeted disruption assay. eGFP fluorescence is disrupted by CRISPR targeting followed by error-prone NHEJ-mediated repair resulting in frameshift mutations that disrupt the coding sequence, resulting in loss of fluorescence. ( c ) Microscope images demonstrating successful CRISPR targeting by U6 or H1 promoter-expressed gRNAs. H7 ES cells were stained and colonies were visualized to show nuclei (left, magenta), eGFP fluorescence (middle, green) and merged images (right) indicating areas of GFP fluorescence mosaicism in the colony. To the right is shown the quantification of eGFP fluorescence loss by flow cytometry for the respective constructs. Below is a higher magnification of an H7 colony targeted by an H1-expressed gRNA showing expression mosaicism. Scale bar, 50 μM. ( d ) Surveyor assay-based quantitation of the frequency of NHEJ. Bioanalyzer gel image depicting control (first lane), U6-expressed gRNA (second lane), H1-expressed gRNA (third lane) and marker (fourth lane). The % indel (as calculated by the fraction of uncut (u) to cut (c) bands) is indicated below. Full size image To confirm and broaden these results with another cell line, we targeted a GFP-expressing human embryonic kidney-293 cell line expressing GFP at the same locus with the same gRNA constructs as above. By Surveyor analysis, we detected a range of efficiencies varying by promoter type and targeting location ( Fig. 1d ; Supplementary Fig. 1 ). Using unmodified IMR90.4-induced pluripotent cells, we also confirmed the ability to modify an endogenous gene by targeting the AAVS-1 locus within the intronic region of the PPP1R12C gene. Targeted cleavage from H1- and U6-driven gRNAs were observed with comparable efficiencies as measured by the Surveyor assay ( Supplementary Fig. 2 ). An expanded CRISPR-targeting space To determine the potential increase in targeting space, we performed bioinformatic analysis to determine the available CRISPR sites in the human genome. While AN 19 NGG sites might be predicted to occur roughly at the same frequently as GN 19 NGG sites, we found that they are actually 15% more common ( Fig. 2 ; Supplementary Fig. 3 ); thus changing specificity from GN 19 NGG to RN 19 NGG more than doubles the number of available sites. With a few exceptions, (chr16, chr17, chr19, chr20 and chr22) AN 19 NGG sites are present at higher frequencies than GN 19 NGG sites on each chromosome. To compare the average genome-wide targeting densities, we calculated the mean distances between adjacent CRISPR sites in the genome for GN 19 NGG (59 bp), AN 19 NGG (47 bp) and RN 19 NGG sites (26 bp) ( Fig. 2b ). In addition, AN 19 NGG sites were even more enriched at relevant regions of targeting in the human genome. We found a 20% increase in AN 19 NGG sites in human genes, and a 21% increase at disease loci obtained from the OMIM database ( Fig. 2c ). We also examined 1,165 micro RNA genes from the human genome and found that 221 of these genes could be targeted through one or more AN 19 NGG sites, but not through a GN 19 NGG site (data not shown). Given that the efficiency of homologous recombination negatively correlates with increasing distance from cut sites, the increase in CRISPR-targeting sites by the use of the H1 promoter should facilitate more precise genomic targeting and mutation correction [24] . 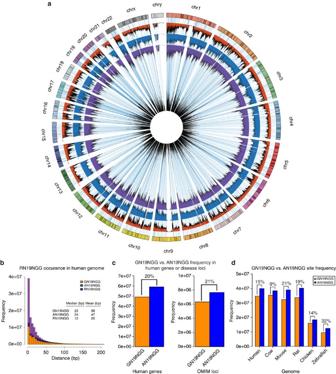Figure 2: Bioinformatics analysis of GN19NGG and AN19NGG sites in the genome. (a) Circos plot depicting the frequency of CRISPR sites in the human genome. The outside circle depicts the human chromosome ideograms. Moving inwards, GN19NGG (orange), AN19NGG (blue) and RN19NGG (purple) CRISPR sites frequency is indicated along the chromosomes. Plotted inside the circle is the human exon density (black), and OMIM disease loci (blue). (b) Frequency and distance between of CRISPR sites in the genome. Barplot of the frequency and distance of adjacent GN19NGG (orange), AN19NGG (blue) sites in the genome. The mean and median values are inset within the plot including RN19NGG sites. (c) Barplot quantification of GN19NGG versus AN19NGG site frequency at human genes (left) or OMIM disease loci (right). (d) Barplot quantifying the GN19NGG versus AN19NGG frequency in six genomes: human, cow, mouse, rat, chicken and zebrafish. Figure 2: Bioinformatics analysis of GN 19 NGG and AN 19 NGG sites in the genome. ( a ) Circos plot depicting the frequency of CRISPR sites in the human genome. The outside circle depicts the human chromosome ideograms. Moving inwards, GN 19 NGG (orange), AN 19 NGG (blue) and RN 19 NGG (purple) CRISPR sites frequency is indicated along the chromosomes. Plotted inside the circle is the human exon density (black), and OMIM disease loci (blue). ( b ) Frequency and distance between of CRISPR sites in the genome. Barplot of the frequency and distance of adjacent GN 19 NGG (orange), AN 19 NGG (blue) sites in the genome. The mean and median values are inset within the plot including RN 19 NGG sites. ( c ) Barplot quantification of GN 19 NGG versus AN 19 NGG site frequency at human genes (left) or OMIM disease loci (right). ( d ) Barplot quantifying the GN 19 NGG versus AN 19 NGG frequency in six genomes: human, cow, mouse, rat, chicken and zebrafish. Full size image As CRISPR technology is increasingly utilized for genomic engineering across a wide array of model organisms, we sought to determine the potential impact of the use of the H1 promoter in other genomes. We carried out this analysis on five other vertebrate genomes that had high genomic conservation at the H1 promoter (mouse; rat; chicken; cow; and zebrafish). In all cases, we found a higher number of AN 19 NGG compared with GN 19 NGG sites: +9% cow; +14% chicken; +19% rat;+21% mouse; and+32% zebrafish ( Fig. 2c ). One explanation for this prevalence could be due to the higher AT content ( Supplementary Fig. 4 ). In the human genome, normalizing the GN 19 NGG and AN 19 NGG site occurrences to AT content brings the frequencies closer to parity, although this does not hold true for all genomes ( Supplementary Fig. 4a,f ). Nevertheless, this demonstrates the utility of using the H1 promoter, which more than doubles the currently available CRISPR-targeting space in the human genome, and similarly in all other genomes tested. Targeting endogenous sites with the H1 promoter construct We next sought to demonstrate the ability to target an AN 19 NGG site in an endogenous gene with the H1 promoter construct. Using H7 cells, we targeted the second exon of the MERTK locus, a gene involved with phagocytosis in the retinal pigment epithelium and macrophages and that when mutated causes retinal degeneration [25] ( Fig. 3a,b ). To estimate the overall targeting efficiency, we harvested genomic DNA from a population of cells that were electroporated, and performed the Surveyor assay. We amplified the region surrounding the target sites with two independent PCR reactions and calculated a 9.5 and 9.7% indel frequency ( Fig. 3b ). Next, 42 randomly chosen clones were isolated and tested for mutation by Surveyor analysis (data not shown). Sequencing revealed that 7/42 (16.7%) harboured mutations clustering within 3–4 nucleotides upstream of the target PAM site. Clones (6/7) had unique mutations (1 clone was redundant) and 3 of these were bi-allelic frame-shift mutations resulting in a predicted null MERTK allele that was confirmed by western blot analysis ( Fig. 3c,d ). Taken together, these results demonstrate the ability to effectively target an AN 19 NGG site located at an endogenous locus. 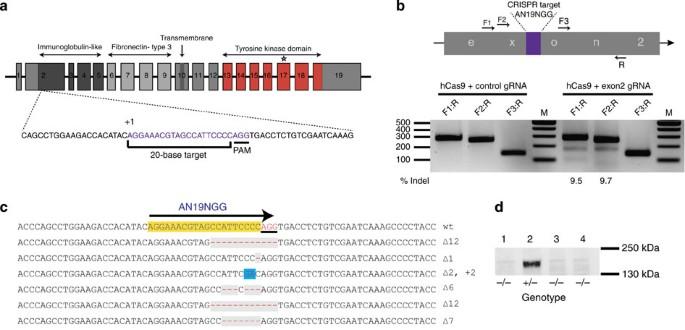Figure 3: CRISPR targeting of AN19NGG at an endogenous gene (MERTK) in H7 ES cells. (a) Schematic diagram of the MERTK locus and various protein domains. Target site in exon 2 is shown below in larger scale, indicating the CRISPR AN19NGG target site. (b) Quantification of CRISPR targeting at exon2 by the Surveyor assay. The CRISPR site in exon 2 is depicted above, with the various primers (arrows) used in the Surveyor assay; both F1:R1 and F2:R2 span the target site, while the control PCR product, F3:R3, is just outside the target site. The gel from the Surveyor assay is shown below with the three control products shown on the left, and targeting is shown on the right. Below the % indel frequency is indicated. (c) Sanger sequencing of mutant lines. Clonal lines were isolated and sequenced indicating that CRISPR targeting at the AN19NGG sites resulted in mutagenesis at this region. The aligned chromatograms show the six unique mutations that were cloned. (d) Western blot analysis for Mertk expression in H7-derrived retinal pigment epithelium cells. Lanes 1, 3 and 4 indicate knockout lines and lane 2 indicates expression from heterozygous line. Rabbit monoclonal anti-MERTK IgG: Abcam ab52968 (1:10,000). Figure 3: CRISPR targeting of AN 19 NGG at an endogenous gene (MERTK) in H7 ES cells. ( a ) Schematic diagram of the MERTK locus and various protein domains. Target site in exon 2 is shown below in larger scale, indicating the CRISPR AN 19 NGG target site. ( b ) Quantification of CRISPR targeting at exon2 by the Surveyor assay. The CRISPR site in exon 2 is depicted above, with the various primers (arrows) used in the Surveyor assay; both F1:R1 and F2:R2 span the target site, while the control PCR product, F3:R3, is just outside the target site. The gel from the Surveyor assay is shown below with the three control products shown on the left, and targeting is shown on the right. Below the % indel frequency is indicated. ( c ) Sanger sequencing of mutant lines. Clonal lines were isolated and sequenced indicating that CRISPR targeting at the AN 19 NGG sites resulted in mutagenesis at this region. The aligned chromatograms show the six unique mutations that were cloned. ( d ) Western blot analysis for Mertk expression in H7-derrived retinal pigment epithelium cells. Lanes 1, 3 and 4 indicate knockout lines and lane 2 indicates expression from heterozygous line. Rabbit monoclonal anti-MERTK IgG: Abcam ab52968 (1:10,000). Full size image To quantitatively determine the extent of off-targeting that occurred from the GFP gRNA constructs, we used Surveyor analysis to examine three genomic loci that were bioinformatically predicted to be off-target sites (GFP_11-33, GFP_219-197 and GFP_315-293). Two of these constructs (GFP_219-197 and GFP_315-293) were GN 19 NGG target sites, allowing for expression with both promoters. One (GFP_11-33), an AN 19 NGG site, was expressed from the U6 promoter by appending a 5′-G nucleotide. In all three off-target loci we examined, we were unable to detect any off-target cleavage (data not shown). However, the lack of detectable off-targets could result from our initial selection of the GFP gRNA targets, in which sites were selected based upon low homology to other genomic loci. Thus, we reasoned that a more stringent challenge would be to compare gRNA expression from H1 and U6 promoters at targeting sites specifically known to elicit high levels of off-target hits [26] , [27] , [28] . Furthermore, the 5′ nucleotide flexibility of the H1 promoter allowed for a direct comparison of identical gRNAs targeting GN 19 NGG sites between U6 and H1 promoters, and we tested two sites previously reported from Fu et al. [26] : VEGFA site 1 (T1) and VEGFA site 3 (T3) ( Table 1 ; Supplementary Fig. 5 ) [26] , [28] . An additional benefit of the H1 promoter over the U6 promoter may be in increasing specificity by reducing spurious cleavage. Because increased gRNA and Cas9 concentrations have been shown to result in increased off-target hits [26] , [27] , [29] , we reasoned that the lower gRNA expression level from the H1 promoter [30] , [31] , [32] might also reduce off-target effects. Using quantitative (q) reverse transcriptase (RT)-PCR, we tested the levels of the VEGFA-T1 gRNA from either the H1 and U6 promoter, confirming the reduced level of expression of the gRNA ( Supplementary Fig. 5a ). For the VEGFA T1 site, we tested the efficiency of cutting at the on-target loci, as well as four off-target loci. In comparison with the U6 promoter, cutting at the on-target loci was comparable or slightly reduced; however, the H1 promoter-expressed gRNAs were notable more stringent at the examined off-target loci indicating greater specificity (off-target 1: 8 versus 25%; off-target 2: undetectable versus 20%; and off-target 4: 9 versus 26%) ( Table 1 ; Supplementary Fig. 5 ). We detected equal targeting between the two promoter constructs at the VEGFA T3 site (26%), but again, lower levels of off-target cutting with the H1 promoter ( Table 1 ; Supplementary Fig. 5 ). While further studies on H1 and U6 promoters expressed gRNAs need to be performed, our data suggest greater specificity from H1-expressed gRNAs. Table 1 Frequency of indels induced at on-target and off-target sites by U6- or H1-expressed gRNAs. Full size table Accumulating evidence for S. pyogenes Cas9 targeting in vitro and in vivo , indicates that the Cas9:gRNA recognition extends throughout the entire 20-base pair targeting site. First, in testing >10 12 distinct variants for gRNA specificity in vitro , one study found that the +1 nucleotide plays a role in target recognition. Furthermore, positional specificity calculations from this data show that the 5′ nucleotide contributes a greater role in target recognition than its 3′ neighbour, indicating that the ‘seed’ model for CRISPR specificity might overly simplify the contribution of PAM-proximal nucleotides [27] . Second, alternative uses such as CRISPR interference, which repurposes the CRISPR system for transcriptional repression, found that 5′ truncations in the gRNA severely compromised repression, and 5′ extensions with mismatched nucleotides—such as mismatched G bases for U6 expression—also reduce the repression efficiency, suggesting that both length (20 nt) and 5′ nucleotide context are important for proper Cas9 targeting [24] , [33] , [34] , [35] , [36] . Finally, crystal structure data further supports the experimental data and importance of the 5′ nucleotide in Cas9, as significant contacts are made with the 5′ nucleotide of the gRNA and 3′ end of the target DNA [37] , [38] . For increased targeting space, the use of alternate Cas9 proteins has been shown to be effective, as in Neisseria meningitidis and S. thermophilus , yet PAM restrictions from other type II systems reported, so far have more stringent requirements and therefore reduce the sequence space available for targeting when used alone (data not shown and refs 11 , 17 ). In contrast, modified gRNA expression by use of the H1 promoter would be expected to greatly expand the targeting repertoire with any Cas9 protein irrespective of PAM differences. When we quantitated the respective gRNAs targets for orthologous Cas9 proteins (AN 23 NNNNGATT versus GN 23 NNNNGATT for N. meningitides and AN 17 NNAGAAW versus GN 17 NNAGAAW for S. thermophilus ), we found a 64 and 69% increase in the gRNA sites with a 5′-A nucleotide, indicating an even greater expansion of targeting space through use of the H1 promoter with alternate Cas9 proteins ( Supplementary Table 1 ). As suggested in plants, use of different promoters can expand the frequency of CRISPR sites. While the U6 promoter is restricted to a 5′ guanosine nucleotide, the U3 promoter from rice is constrained to a 5′ adenosine nucleotide further highlighting the need for different promoters in different systems to increase targeting space [36] . Conveniently, sole use of the H1 promoter can be leveraged to target AN 19 NGG and GN 19 NGG sites (and possibly CN 19 NGG or TN 19 NGG sites [39] ) via a single promoter system ( Supplementary Fig. 6 ). This in turn can be employed to expand targeting space of both current and future Cas9 variants with altered sites restrictions. Similarly with ZFN or TALEN technologies, one approach to mitigate potential off-target effects might be to employ cooperative offset nicking with the Cas9 mutant (D10A or H840A) [24] , [35] . This requires identification of two flanking CRISPR sites, oriented on opposing strands, and within ~20 bp of the cut site [24] , and thus the additional targeting density provided by AN 19 NGG sites would be expected to augment this approach. An added benefit over the U6 promoter may also be to reduce spurious cleavage; as several groups have reported that increased gRNA and Cas9 concentrations correlate with an increase in the propensity for off-target mutations [26] , [27] , [29] , the lower level of expression provided by the H1 promoter may result in reduced off-target cutting. With enhanced CRISPR targeting through judicious site selection, improved Cas9 variants, optimized gRNA architecture or additional cofactors, an increase in specificity throughout the targeting sequence will likely result, placing greater importance on the identity of the 5′ nucleotide. As a research tool, this will allow for greater manipulation of the genome while minimizing confounding mutations, and for future clinical applications, high targeting densities coupled with high-fidelity target recognition will be paramount to delivering safe and effective therapeutics. Plasmid construction To generate the H1 gRNA-expressing construct, overlapping oligos were assembled to create the H1 promoter fused to the 76-bp gRNA scaffold and pol III termination signal. In between the H1 promoter and the gRNA scaffold, a Bam HI site was incorporated to allow for the insertion of targeting sequence. The H1::gRNA scaffold::pol III terminator sequence was then TOPO cloned into pCR4-Blunt (Invitrogen), and sequenced verified; the resulting vector is in the reverse orientation (see below). To generate the various gRNAs used in this study ( Supplementary Table 2 ), overlapping oligos were annealed and amplified by PCR using two-step amplification Phusion Flash DNA polymerase (Thermo Scientific), and subsequently purified using Carboxylate-Modified Sera-Mag Magnetic Beads (Thermo Scientific) mixed with 2 × volume 25% polyethylene glycol and 1.5 M NaCl. The purified PCR products were then resuspended in H 2 O and quantitated using a NanoDrop 1000. The gRNA-expressing constructs were generated using the Gibson assembly [40] (NEB) with slight modifications for either the AflII-digested plasmid (Addgene #41824) for U6 expression, or Bam HI digestion of plasmid just described for H1 expression. The total reaction volume was reduced from 20 to 2 μl. Cell culture The hESC line H7 and IMR-90.4 iPS cells (WiCell) were maintained by clonal propagation on growth factor-reduced Matrigel (BD Biosciences) in mTeSR1 medium (Stem Cell Technologies), in a 10% CO 2 /5% O 2 incubator according to previously described protocols [41] , [42] . For passaging, hPSC colonies were first incubated with 5 μM blebbistatin (Sigma) in mTesR1, and then collected after 5–10 min treatment with Accutase (Sigma). Cell clumps were gently dissociated into a single-cell suspension and pelleted by centrifugation. Thereafter, hPSCs were resuspended in mTeSR1 with blebbistatin and plated at ~1,000–1,500 cells cm −2 . Two days after passage, medium was replaced with mTeSR1 (without blebbistatin) and changed daily. Human embryonic kidney cell line 293T (Life Technologies, Grand Island, NY, USA) was maintained at 37 °C with 5% CO 2 /20% O 2 in Dulbecco’s modified Eagle’s medium (Invitrogen) supplemented with 10% fetal bovine serum (Gibco) and 2 mM GlutaMAX (Invitrogen). Gene targeting of H7 cells hESC cells were cultured in 10 μM Rho Kinase inhibitor (DDD00033325 EMD Millipore) 24 h before electroporation. Electroporation were performed using the Neon kit (Invitrogen), according to the manufacturer’s instruction. Briefly, on the day of electroporation, hESC were digested with Accutase (Sigma) for 1–2 min until colonies lifted. Importantly, colonies were not dissociated into a single-cell suspension. After colonies were harvested, wet pellets were kept on ice for 15 min, and then resuspended in electroporation buffer containing gene-targeting plasmids. Electroporation parameters were as following: voltage: 1,400 ms; interval: 30 ms; 1 pulse. Following electroporation, cell colonies were slowly transferred to mTeSR1 medium containing 10 μM Rho Kinase inhibitor, and then kept at room temperature for 20 min before plating on Matrigel-coated dishes and further cultured. For analysis of clonally derived colonies, electroporated hESC were grown to sub-confluence, passaged as described in the previous paragraph and plated at a density of 500 cells per 35 mm dish. Subsequently, single colonies were isolated by manual picking and further cultured. For 293T cell transfection, ~100,000 cells per well were seeded in 24-well plates (Falcon) 24 h before transfection. Cells were transfected in quadruplicates using the Lipofectamine LTX Plus Reagent (Invitrogen) according to the manufacturer’s recommended protocol. For each well of a 24-well plate, 400 ng of the Cas9 plasmid and 200 ng of the gRNA plasmid were mixed with 0.5 μl of Plus Reagent and 1.5 μl of Lipofectamine LTX reagent. Generation of constitutively expressed GFP ESC lines The H7 human ESC line (WiCell) was maintained in mTeSR1 (Stem Cell Technologies) media on Matrigel substrate. Prior to cell passaging, cells were subjected to a brief pre-treatment with blebbistatin (>5 min) to increase cell viability, treated with Accutase for 7 min, triturated to a single-cell suspension, quenched with an equal volume of mTesR1, pelleted at 80 g for 5 min and resuspended in mTesR1 containing blebbistatin. Cells (1 × 10 6 ) were pelleted, media carefully removed and cells placed on ice for 10–15 min. Ten microgram of AAV-CAGGS-EGFP donor vector (Addgene; #22212) containing homology to the AAVS-1 safe-harbour locus, plus 5 μg each of hAAVS1 1R+L TALENs (Addgene # 35431 and 35432 (refs 23 , 43 )) in R-buffer were electroporated with a 100 μl tip-type using the Neon Transfection System (Life Technologies) with the following parameters: 1,500 V, 20 ms pulse and 1 pulse. Cells were then added gently to 1 ml of medium and incubated at room temperature for 15 min and then plated onto Matrigel-coated 35 mm dishes containing mTeSR and 5 μM blebbistatin. After 2 days, cells were seeded at a density of 1 × 10 4 after which time-stable clonal sublines were manually selected with a fluorescence equipped Nikon TS100 epifluorescence microscope. Surveyor analysis and quantification of genome modification For Surveyor analysis, genomic DNA was extracted by resuspending cells in QuickExtract solution (Epicentre), incubating at 65 °C for 15 min, and then at 98 °C for 10 min. The extract solution was cleaned using DNA Clean and Concentrator (Zymo Research) and quantitated by NanoDrop. The genomic region surrounding the CRISPR target sites was amplified from 100 ng of genomic DNA using Phusion DNA polymerase (NEB). Multiple independent PCR reactions were pooled and purified using Qiagen MinElute Spin Column following the manufacturer’s protocol. An 8 μl volume containing 400 ng of the PCR product in 12.5 mM Tris-HCl (pH 8.8), 62.5 mM KCl and 1.875 mM MgCl 2 was denatured and slowly re-annealed to allow for the formation of heteroduplexes: 95 °C for 10 min, 95 °C to 85 °C ramped at −1.0 °C s −1 , 85 °C for 1 s, 85 °C to 75 °C ramped at −1.0 °C s −1 , 75 °C for 1 s, 75 °C to 65 °C ramped at −1.0 °C s −1 , 65 °C for 1 s, 65 °C to 55 °C ramped at −1.0 °C s −1 , 55 °C for 1 s, 55 °C to 45 °C ramped at −1.0 °C s −1 , 45 °C for 1 s, 45 °C to 35 °C ramped at −1.0 °C s −1 , 35 °C for 1 s, 35 °C to 25 °C ramped at −1.0 °C s −1 , and then held at 4 °C. One microlitre of Surveyor Enhancer and 1 μl of Surveyor Nuclease (Transgenomic) were added to each reaction, incubated at 42 °C for 60 min, after which, 1 μl of the stop solution was added to the reaction. One microlitre of the reaction was quantitated on the 2100 Bioanalyzer using the DNA 1000 chip (Agilent). For gel analysis, 2 μl of 6 × loading buffer (NEB) was added to the remaining reaction and loaded onto a 3% agarose gel containing ethidium bromide. Gels were visualized on a Gel Logic 200 Imaging System (Kodak), and quantitated using ImageJ v. 1.46. NHEJ frequencies were calculated using the binomial-derived equation: % gene modification= ; where the values of ‘ a ’ and ‘ b ’ are equal to the integrated area of the cleaved fragments after background subtraction and ‘ c ’ is equal to the integrated area of the un-cleaved PCR product after background subtraction [44] . Flow cytometry Following blebbistatin treatment, sub-confluent hESC colonies were harvested by Accutase treatment, dissociated into a single-cell suspension and pelleted. Cells were then resuspended in Live Cell Solution (Invitrogen) containing Vybrant DyeCycle ruby stain (Invitrogen) and analysed on an Accuri C6 flow cytometer. Quantitative real-time PCR 293T cells were seeded at 250,000 cells per well in 12-well plates (Falcon) 24 h before transfection. Cells were transfected in triplicate using Lipofectamine LTX with Plus Reagent (Invitrogen) according to the manufacturer’s recommended protocol with a six-dose titration of the gRNA plasmid: 0, 31.25, 62.5, 125, 250 or 500 ng in each well. Forty-eight hours post transfection, total RNA was isolated using RNAzol RT (Molecular Research Center), and purified using Direct-zol RNA MiniPrep (Zymo). Total RNA (500 ng) was double-strand specific dsDNase (ArticZymes; Plymouth Meeting, PA USA) treated to remove residual genomic DNA contamination and reverse transcribed in a 20-μl reaction using Superscript III reverse transcriptase (Invitrogen) following the manufacturer’s recommendations. For each reaction, 0.1 μM of the following oligonucleotides were used to prime each reaction; gRNA scaffold-5′- CTTCGATGTCGACTCGAGTC AAAAAGCACCGACTCGGTGCCAC-3′, U6 snRNA-5′-AAAATATGGAACGCTTCACGAATTTG-3′. The underlined scaffold sequence denotes an anchor sequence added for transcript stability. Each qPCR reaction was carried out in a Bio-Rad CFX 96 real-time PCR machine in a 10-μl volume using the SsoAdvanced Universal SYBR Green Supermix (Bio-Rad) containing 250 nM of oligonucleotide primers and 1 μl of a 1:15 dilution of the RT reaction product from above. Reactions were carried out for 40 cycles with 95 °C denaturation, 54 °C annealing temperature and 60 °C extension steps. The following primers were used for detecting the gRNA and reference gene, respectively: F1for-5′-GTTTTAGAGCTAGAAATAGCAAGTTAA-3′ and guideRNAscaffrev-5′-AAGCACCGACTCGGTGCCAC-3′ and U6snRNAF-5′-CTCGCTTCGGCAGCACATATACT-3′ and U6snRNARev-5′-ACGCTTCACGAATTTGCGTGTC-3′. Relative normalized expression for each gRNA sample and the s.e.m. was calculated using Bio-Rad’s integrated CFX manager software. Bioinformatics To determine all the potential CRISPR sites in the human genome, we used a custom Perl script to search both strands and overlapping occurrences of the 23-mer CRISPR sequence sites GN 19 NGG or AN 19 NGG. To calculate the mean and median distance values, we first defined the predicted CRISPR cut site as occurring between the third and fourth bases upstream of the PAM sequence. After sorting the sequences, we then calculated the distances between all adjacent gRNAs in the genome. This data were imported into R to calculate the mean and median statistical values, and to plot the data. To calculate the mean density, the gRNA cut sites were binned across the genome and calculated for the frequency of occurrences. These data were plotted in R using the ggplot2 package, or used Circos to generate a circular plot [45] . To calculate the occurrences in human genes or at disease loci, we used BEDTools utility IntersectBED [46] to find the occurrence of overlaps with either a RefSeq BED file retrieved from the UCSC Genome Browser or a BED file from OMIM (Online Mendelian Inheritance in Man, OMIM. McKusick-Nathans Institute of Genetic Medicine, Johns Hopkins University (Baltimore, MD, USA), 2013. World Wide Web URL: http://omim.org/ ). As a reference, on average, TALEN targeting sites are estimated to occur every 35 base pairs and ZFN sites occur every couple hundred base pairs [3] , [47] . The genomes used in this study were human (hg19), mouse (mm10), rat (rn5), cow (bosTau7), chicken (galGal4), zebrafish (dr7), drosophila (dm3), C. elegans (ce10) and S. cerevisiae (sacCer3). How to cite this article: Ranganathan, V. et al. Expansion of the CRISPR–Cas9 genome targeting space through the use of H1 promoter-expressed guide RNAs. Nat. Commun. 5:4516 doi: 10.1038/ncomms5516 (2014).